Large spin-orbit coupling in carbon nanotubes It has recently been recognised that the strong spin-orbit interaction present in solids can lead to new phenomena, such as materials with non-trivial topological order. Although the atomic spin-orbit coupling in carbon is weak, the spin-orbit coupling in carbon nanotubes can be significant due to their curved surface. Previous works have reported spin-orbit couplings in reasonable agreement with theory, and this coupling strength has formed the basis of a large number of theoretical proposals. Here we report a spin-orbit coupling in three carbon nanotube devices that is an order of magnitude larger than previously measured. We find a zero-field spin splitting of up to 3.4 meV, corresponding to a built-in effective magnetic field of 29 T aligned along the nanotube axis. Although the origin of the large spin-orbit coupling is not explained by existing theories, its strength is promising for applications of the spin-orbit interaction in carbon nanotubes devices. In solids, spin-orbit coupling has recently become a very active topic, in particular in the context of its role in a new class of materials with a non-trivial topological order [1] , [2] , [3] , and its use to enable new control techniques in solid-state qubits based on manipulating spins with electric fields [4] , [5] . Owing to the low atomic number of the carbon nucleus, the spin-orbit interaction in carbon materials is, in general, weak. An example of this is flat graphene, in which intrinsic spin-orbit effects are expected to appear at energy scales of only 1 μeV (10 mK) [6] , [7] . In carbon nanotubes, however, the curvature of the surface breaks a symmetry that is present in graphene. This broken symmetry enhances the intrinsic spin-orbit coupling in carbon nanotubes compared with flat graphene, with theoretical estimates predicting splittings on the order of 100 μeV, an energy scale easily accessible in transport measurements at dilution refrigerator temperatures, and recently observed in experiments [8] , [9] , [10] , [11] . Experiments so far have reported spin-orbit splittings typically in the range of hundreds of μeV, and which were reasonably consistent with theoretical predictions. Since it was first observed experimentally, the spin-orbit interaction in carbon nanotubes has attracted significant theoretical attention, and has been the basis of a large number of theoretical proposals. Recent calculations predict that it enables fast electrical spin manipulation in carbon nanotube spin qubits [12] , [13] , that it can couple to the phase of Josephson supercurrents through Andreev bound states in nanotube superconducting junctions [14] , [15] , that it allows the spin to couple to the high quality vibrational modes of nanotubes [16] , [17] and that it could be interesting for the study of topological liquids and Majorana bound states [18] , [19] , [20] , [21] , [22] . These many exciting proposed applications could potentially benefit from a stronger spin-orbit coupling. Here, we present measurements of three carbon nanotube devices which have spin-orbit couplings an order of magnitude larger than that predicted by theory. We observe the spin-orbit coupling by measuring the magnetic field dependence of the ground states of clean carbon nanotube quantum dots in the few-electron and few-hole regime [23] . We use a Dirac-point crossing at a low magnetic field as a tool for distinguishing orbital-type coupling [24] , [25] , [6] from the recently predicted Zeeman-type coupling [26] , [27] , [28] . Although it is not understood why the spin-orbit coupling we observe is so much larger than that predicted by tight-binding calculations, its large magnitude is attractive for implementing the theoretical proposals for using the carbon nanotube spin-orbit coupling for a wide range of new experiments. Spin-orbit coupling in a few electron nanotube quantum dot The devices are made using a fabrication technique in which the nanotube is deposited in the last step of the fabrication. 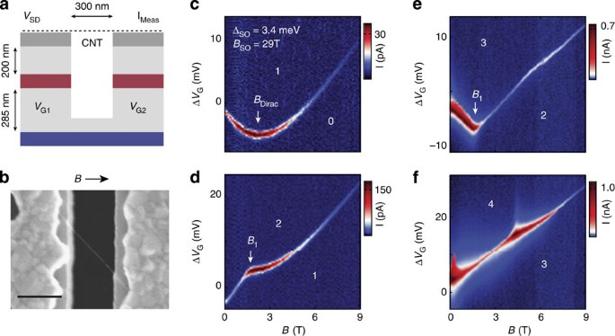Figure 1: A 29 T spin-orbit magnetic field in a carbon nanotube. (a) A schematic of device 1. (b) A scanning electron microscope (SEM) image of device 1. Scale bar, 300 nm. Scale bar, 300 nm. The arrow indicates the direction of the applied magnetic fieldB. (c–f) Magnetic field dependence of the Coulomb peak positions of the first four electrons in the device.VSD=200 μV in (c,d) andVSD=150 μV in (e,f). ΔVGcorresponds to a small offset in gate voltage used to track the Coulomb peaks as a function of magnetic field. The crossing of the Dirac point reverses the sign of the orbital magnetic moment of the lower energy valley at a fieldBDirac=2.2 T. Without spin-orbit coupling, the first two electrons would both occupy the valley with the decreasing orbital energy, and would result in a downwards slope in both (c,d) at fields belowBDirac. Here, the second electron, (d), instead occupies a valley with increasing orbital energy, a unique signature of the nanotube spin-orbit coupling, up to a fieldB1=1.6 T. From the ground state energies extracted from the Coulomb peak positions,Fig. 3(a), we obtain a spin-orbit splitting ΔSO=3.4±0.3 meV, corresponding to a built-in spin-orbit magnetic fieldBSO=29 T seen by the electron spin. The sharp kinks atB1in (d,e) imply weak valley mixing: we estimate ΔKK′~0.1 meV. Figure 1a shows a schematic of a single quantum dot device with three gates. Figure 1b shows a scanning electron microscope image of device 1, taken after all measurements were completed. Similar to previous reports [23] , we are able to tune the device to contain only a single electron (see Supplementary Note 1 and Supplementary Figs S1,S2 ). An external magnetic field is applied in-plane, perpendicular to the trench. As we do not control the direction of the growth process, this magnetic field often has a misalignment to the nanotube, but still contains a large component parallel to the nanotube axis. All measurements were performed in a dilution refrigerator with an electron temperature of 100 mK. Figure 1: A 29 T spin-orbit magnetic field in a carbon nanotube. ( a ) A schematic of device 1. ( b ) A scanning electron microscope (SEM) image of device 1. Scale bar, 300 nm. Scale bar, 300 nm. The arrow indicates the direction of the applied magnetic field B . ( c–f ) Magnetic field dependence of the Coulomb peak positions of the first four electrons in the device. V SD =200 μV in ( c , d ) and V SD =150 μV in ( e , f ). Δ V G corresponds to a small offset in gate voltage used to track the Coulomb peaks as a function of magnetic field. The crossing of the Dirac point reverses the sign of the orbital magnetic moment of the lower energy valley at a field B Dirac =2.2 T. Without spin-orbit coupling, the first two electrons would both occupy the valley with the decreasing orbital energy, and would result in a downwards slope in both ( c , d ) at fields below B Dirac . Here, the second electron, ( d ), instead occupies a valley with increasing orbital energy, a unique signature of the nanotube spin-orbit coupling, up to a field B 1 =1.6 T. From the ground state energies extracted from the Coulomb peak positions, Fig. 3 ( a ), we obtain a spin-orbit splitting Δ SO =3.4±0.3 meV, corresponding to a built-in spin-orbit magnetic field B SO =29 T seen by the electron spin. The sharp kinks at B 1 in ( d , e ) imply weak valley mixing: we estimate Δ KK′ ~0.1 meV. Full size image In Fig. 1c–f , we show the magnetic field dependence of the Coulomb peaks of the first four electrons in a carbon nanotube quantum dot in device 1. In the few electron regime, we estimate the single-particle level spacing of the quantum dot to be Δ E SP =11 meV (see Supplementary Fig. S3 ). Note that similar to recent reports [29] , this device exhibits a crossing of the Dirac point at an anomalously low magnetic field, causing a reversal of the orbital magnetic moment of one of the valleys at B Dirac =2.2 T (see Fig. 2c–f ). The low B Dirac indicates a small shift of the k ┴ quantisation line from the Dirac point ( Fig. 2a ), and would predict a small electronic bandgap contribution from the momentum k ┴ of the electronic states around the nanotube circumference: meV. We describe a nanotube with a low Dirac-field crossing as ‘nearly metallic’, as the k ┴ quantisation line nearly passes through the Dirac point. The bandgap in our device does not vanish at B Dirac , as would be expected, but instead retains a large residual contribution meV, similar to previous reports [29] . It has been suggested that this residual energy gap could arise from a Mott-insulating state, although its exact origin remains a topic of investigation that we will not address here. This low Dirac-field crossing does not affect the spin-orbit spectra we observe, and will later provide a unique signature for distinguishing orbital [24] , [25] , [6] from Zeeman- [26] , [27] , [28] type coupling. We first focus on the behaviour at magnetic fields below B Dirac . 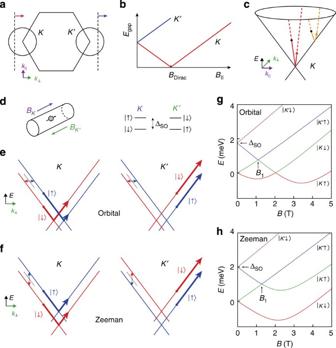Figure 2: Spin-orbit coupled states in a nearly-metallic nanotube. (a) The two nanotube valleys (KandK′) arise from the intersection of thek┴quantisation lines (dashed) with the Dirac cones of the graphene bandstructure. A magnetic field applied parallel to the nanotube axis shifts both quantisation lines horizontally, reducing the bandgap in oneKpoint and increasing it for the other, illustrated in (b). At a sufficiently large magnetic fieldBDirac, one valley (red line) crosses the Dirac point, after which the orbital magnetic moment changes sign. (c) With=0, the lowest energy state in the conduction band would follow a v-shape with a sharp kink atBDirac(red line inb,c). A finitefrom confinement in the axial direction results instead in a hyperbolic shape (orange line inc). (d) The spin-orbit interaction in the nanotube results in an internal magnetic field aligned along the nanotube axis whose direction depends on the valley the electron occupies. (e) In the orbital-type spin-orbit coupling24,25,6, this magnetic field results in a spin-dependent shift ofk┴, while the Zeeman-type coupling, (f), gives a valley dependent vertical shift in energy26,27,28. (g,h) Calculated energy spectrum of the first shell for a purely orbital-type coupling, (g), and a purely Zeeman-type coupling, (h), with parameters chosen to illustrate the difference between the two types of spectra. Colours indicate the ground state energies of the four electrons that would fill the shell. In (g), electrons experience a spin-dependentk┴shift, resulting in two separate Dirac crossings10, an effect absent in (h). Figure 2: Spin-orbit coupled states in a nearly-metallic nanotube. ( a ) The two nanotube valleys ( K and K ′) arise from the intersection of the k ┴ quantisation lines (dashed) with the Dirac cones of the graphene bandstructure. A magnetic field applied parallel to the nanotube axis shifts both quantisation lines horizontally, reducing the bandgap in one K point and increasing it for the other, illustrated in ( b ). At a sufficiently large magnetic field B Dirac , one valley (red line) crosses the Dirac point, after which the orbital magnetic moment changes sign. ( c ) With =0, the lowest energy state in the conduction band would follow a v-shape with a sharp kink at B Dira c (red line in b , c ). A finite from confinement in the axial direction results instead in a hyperbolic shape (orange line in c ). ( d ) The spin-orbit interaction in the nanotube results in an internal magnetic field aligned along the nanotube axis whose direction depends on the valley the electron occupies. ( e ) In the orbital-type spin-orbit coupling [24] , [25] , [6] , this magnetic field results in a spin-dependent shift of k ┴ , while the Zeeman-type coupling, ( f ), gives a valley dependent vertical shift in energy [26] , [27] , [28] . ( g , h ) Calculated energy spectrum of the first shell for a purely orbital-type coupling, ( g ), and a purely Zeeman-type coupling, ( h ), with parameters chosen to illustrate the difference between the two types of spectra. Colours indicate the ground state energies of the four electrons that would fill the shell. In ( g ), electrons experience a spin-dependent k ┴ shift, resulting in two separate Dirac crossings [10] , an effect absent in ( h ). Full size image The unambiguous signature of the nanotube spin-orbit interaction can be seen by comparing the low magnetic field behaviour in Fig. 1c . Owing to the opposite direction of circulation of the electronic states about the nanotube circumference, the bandgap of the K and K ′ valleys both change in the presence of a parallel magnetic field [30] , [31] . The bandgap in one valley increases and the other decreases, both with a rate given by dE / dB =2 μ orb , where μ orb =dev F┴ /4 ( μ orb ~220 μeV/T for d =1 nm). In the absence of spin-orbit coupling, the first two electrons would both occupy the valley with lower energy, and thus the first two ground states would both shift down in energy with magnetic field. In Fig. 1c , we observe a different behaviour: in particular, at low magnetic fields, the second electron instead occupies the valley that is increasing in energy with magnetic field. The occupation of the ‘wrong valley’ by the second electron is a result of the nanotube spin-orbit interaction [8] : the spin-orbit coupling in nanotubes results in an effective magnetic field aligned along the nanotube axis, which points in opposite directions for the K and K ′ valleys ( Fig. 2d ). This magnetic field produces a spin splitting Δ SO for the two spin species in the same valley. In an external magnetic field, the second electron then enters the ‘wrong’ valley, and persists there until the energy penalty for this exceeds Δ SO . In device 1, from the extract ground-state spectra shown in Fig. 3(a) , we find a Δ SO =3.4±0.3 meV. In addition to the ground state measurements, states consistent with such a splitting have been observed in finite bias excited state spectroscopy (see Supplementary Figs S3,S4 ). We have also observed a large Δ SO =1.5±0.2 meV in a second similar single-dot device (see Supplementary Figs S5–S9 , and Supplementary Note 2 ). 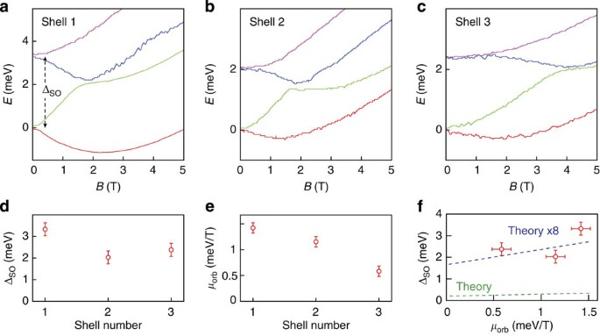Figure 3: Spin-orbit coupling in the first three electronic shells. (a–c) Observed energy spectra of the first 12 electrons in device 1. The spectra exhibits a four-fold shell filling, with the spin-orbit electronic spectrum visible in all three shells. Extracted ΔSOare shown in (d). Comparing with the spectra for the two types of nanotube spin-orbit coupling (Fig. 2g), it is clear the device exhibits a Zeeman-type coupling. Deviations from the model are discussed in the main text. (e)μorbas a function of the shell number. For larger shells, electrons are confined in an electronic level with a larger value of. The correspondingly larger momentum along the nanotube axis decreases the velocity around the nanotube circumference, reducing the orbital magnetic moment11,32. (f) ΔSOas a function ofμorb. The green dashed line shows the maximum spin-orbit coupling expected from theory withαandβfor a 3-nm nanotube (equation 1 together with the scaling ofαwith the magnetic moment). By scaling coefficientsαandβby a factor of 8 (blue line), we can reproduce the order of magnitude of the spin-orbit coupling in our device. Figure 3: Spin-orbit coupling in the first three electronic shells. ( a – c ) Observed energy spectra of the first 12 electrons in device 1. The spectra exhibits a four-fold shell filling, with the spin-orbit electronic spectrum visible in all three shells. Extracted Δ SO are shown in ( d ). Comparing with the spectra for the two types of nanotube spin-orbit coupling ( Fig. 2g ), it is clear the device exhibits a Zeeman-type coupling. Deviations from the model are discussed in the main text. ( e ) μ orb as a function of the shell number. For larger shells, electrons are confined in an electronic level with a larger value of . The correspondingly larger momentum along the nanotube axis decreases the velocity around the nanotube circumference, reducing the orbital magnetic moment [11] , [32] . ( f ) Δ SO as a function of μ orb . The green dashed line shows the maximum spin-orbit coupling expected from theory with α and β for a 3-nm nanotube (equation 1 together with the scaling of α with the magnetic moment). By scaling coefficients α and β by a factor of 8 (blue line), we can reproduce the order of magnitude of the spin-orbit coupling in our device. Full size image Spin-orbit coupling in nearly-metallic carbon nanotubes In Fig. 2 , we show calculated energy levels of a nearly-metallic carbon nanotube including the spin-orbit interaction. In carbon nanotubes, there are two contributions to the spin-orbit coupling, one which we describe as orbital-type coupling, which induces a shift in the k ┴ quantisation line [26] , [27] , [28] and results in an energy shift proportional to the orbital magnetic moment. The second type, which we describe as Zeeman type, shifts only the energy of the electron spin with no shift in k ┴ . The energy and momentum shifts from these couplings are illustrated in Fig. 2e . Combining these two effects, we have the following Hamiltonian for the spin-orbit interaction (equation 71 in 28 ): where S Z is the spin component along the axis of the nanotube, σ 1 leads to a spin-dependent horizontal shift of the dispersion relation along k ┴ that is of opposite sign in different valleys, while τ leads to a spin-dependent vertical shift that is opposite in the two valleys. The first term represents the orbital-type of coupling, while the second represents the Zeeman-type coupling. The coefficients α and β determine the strength of the two types of coupling, with meV nm)/ r at , and meV nm)/ r where θ is the chiral angle of the nanotube wrapping vector [28] , and r is the radius of the nanotube in nanometres. Through the cos(3 θ ) term, is dependent on the chirality of the nanotube, and is maximum for nanotubes with θ =0, corresponding to the zigzag wrapping vector. Direct experimental observation of the Zeeman-type coupling has been, until now, difficult. There have been two reported indications of a Zeeman-type coupling. The first is a different Δ SO for holes and electrons [26] , [27] , which is not present in the orbital-type spin-orbit models [24] , [25] , [6] . Such an asymmetry was observed in the initial experiments by Kuemmeth et al. [8] , and motivated in part the initial theoretical work predicting the Zeeman-type coupling [26] , [27] . The second indication is a scaling of Δ SO over a large number of electronic shells, as seen in recent experiments [11] , from which a small Zeeman-type contribution was extracted. The low Dirac-field crossing in the nearly-metallic carbon nanotubes studied here provides a unique signature that allows us to identify the type of coupling by looking at the energy spectrum of only a single shell. In Fig. 2g , we show the calculated energy spectrum for a nearly-metallic carbon nanotube with purely orbital-type coupling (see Supplementary Note 3 for details of the model). As the orbital-type coupling shifts k ┴ , the spin-up and spin-down states cross the Dirac point at significantly different magnetic fields [10] . For a purely Zeeman-type coupling, Fig. 2h , the two spin states cross the Dirac point at the same magnetic field. By comparing the theoretical predictions in Fig. 2g to the observed energy spectrum extracted from the Coulomb peaks in Fig. 3a , we can clearly identify a Zeeman-type spin-orbit coupling, suggesting that this nanotube has a chiral vector near θ =0. However, the magnitude of the spin-orbit splitting is much larger than that predicted by theory (see Supplementary Table S1 and Supplementary Note 4 for a summary of expected theoretical values and previous experimental observations). One possible origin for the observed discrepancy is an underestimate of the bare atomic spin-orbit coupling parameter from ab-initio calculations, which enters the tight-binding calculations as an empirical input parameter. In Fig. 3 , we show the ground state energies of the first 12 electrons as a function of magnetic field, extracted from the Coulomb peak positions ( Supplementary Fig. S9 ). The ground states energies follow a four-fold periodic shell-filling pattern, with the spin-orbit split energy spectrum reproduced in the second and third electronic shell. In Fig. 3e , we plot the orbital magnetic moment as a function of shell number, including a correction for the angle between the magnetic field and the nanotube axis. As reported previously [32] , the orbital magnetic moment changes with shell number, an effect particularly strong in our device owing to the small k ┴ implied by the low magnetic field Dirac crossing. In Fig. 3f , we plot the observed Δ SO as a function of the orbital magnetic moment, together with the theoretical predictions from equation 1. In the plot, we have included the fact that the orbital coupling coefficient α in equation 1 scales with the orbital magnetic moment [11] . The green dashed line shows the prediction from equation 1 for a nanotube with a 3-nm diameter, emphasising the disagreement between measured and the theoretically predicted values. Also shown is the same prediction with the coefficients scaled by a factor of 8 in order to obtain the order of magnitude of the observed splitting. Note that there are some discrepancies between the energy spectrum extracted from the Coulomb peak positions ( Fig. 3a–c ) and the theoretical spectra presented in Fig. 2 . The first discrepancy is a small curvature of the extracted ground state energies at B <0.15 T in Fig. 3a–c , which we attribute to artifacts from way in which the magnetic field sweeps were performed (see Supplementary Note 5 and Supplementary Fig. S10 ). The second discrepancy is a bending of the extracted energies at B <1.5 T, particularly noticeable in the upper two states of the second and third shells (blue and purple lines in Fig. 3b ), and a resulting suppressed slope for B <1.5 T in these states. Correlated with the gate voltages and magnetic fields where the suppressed slopes occur, we observed a strong Kondo effect present in the odd valleys (see Supplementary Fig. S2 ). Owing to the strong tunnel coupling to the leads, the Kondo current in the valley can persist up to fields of 1.5 T (see Supplementary Fig. S9 ), and is stronger in the higher shells where the tunnel coupling to the leads is larger. The model described in Fig. 2 does not include higher-order effects, such as Kondo correlations, and it seems that it is no able to correctly predict the position of the Coulomb peak in these regions. Qualitatively, the magnetic moments associated with the states appear to be reduced by the strong Kondo effect, although the reason for this is not understood. Note that a suppressed magnetic moment will reduce the apparent spin-orbit splitting, and thus the large spin-orbit splittings reported here represent a lower bound. Large spin-orbit coupling in a nanotube double quantum dot In Fig. 4 , we present data from a third device in a p–n double quantum dot configuration that also exhibits an unexpectedly large spin-orbit coupling (see Supplementary Note 6 and Supplementary Figs S11,S12 for device details and characterization). 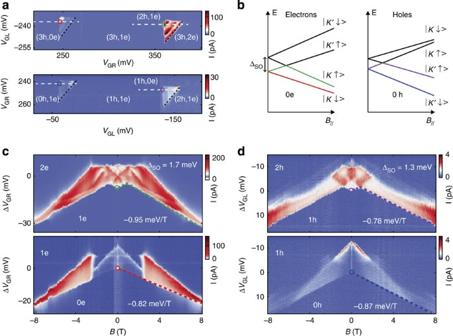Figure 4: Large spin-orbit coupling in a (p,n) double quantum dot. (a) Colour scale plots of the current at a source-drain biasVsd=5 mV andB=0. Black dashed lines indicate the baseline of the triple-point bias triangles. Movement of the tip of the bias triangles (coloured circles) in gate space along line cuts in gate space (white dashed lines) with magnetic field is used in (c,d) to track the ground state energies. (b) Expected energy spectrum for the first shell of electrons and holes including the spin-orbit interaction. (c,d) Magnetic field dependence of line cuts in gate space (white dashed lines ina) for the first two electrons, (c), and holes, (d). Coloured circles indicate positions on the corresponding bias triangles in (a), and the dashed lines indicate the observed magnetic field dependence of the ground states, in good agreement with the spin-orbit spectrum, (b). High magnetic field slopes for the ground state energies are indicated in the figures. We extract spin-orbit splittingsmeV for the first electron shell andmeV for the first hole shell. Excited states inside the bias triangles (colour scale data above dashed lines) exhibit a rich structure as a function magnetic field, which we discuss elsewhere33. Figure 4c show measurements of the ground state energies of the first two electrons and first two holes in the device as a function of parallel magnetic field, measured by tracking the position of a fixed point on the bias triangle in gate space (coloured circles in Fig. 4 a) as a function of magnetic field. The signature of the nanotube spin-orbit interaction can be clearly seen by the opposite slope of the first two electrons (holes) in Fig. 4c ( Fig. 4d ), and is consistent with the carbon nanotube spin-orbit spectrum far from the Dirac crossing, shown in Fig. 4b . The difference in the high magnetic field slopes corresponds to a Zeeman splitting with g ~2, as expected from the spin-orbit spectrum. By calibrating the gate voltage shifts into energy using the size and orientation of the finite bias triangles (see Supplementary Note 6 ), we extract an orbital magnetic moment of μ orb =0.8 meV/T, a spin-orbit splitting meV for the first electron shell, and meV for the first hole shell. Estimating the diameter from the orbital magnetic moment, theory would predict a meV for this device, an order of magnitude below the observed values. Note that device 3 exhibits a large spin-orbit coupling without a low B Dirac , suggesting that these two phenomena are not linked. Figure 4: Large spin-orbit coupling in a (p,n) double quantum dot. ( a ) Colour scale plots of the current at a source-drain bias V sd =5 mV and B =0. Black dashed lines indicate the baseline of the triple-point bias triangles. Movement of the tip of the bias triangles (coloured circles) in gate space along line cuts in gate space (white dashed lines) with magnetic field is used in ( c , d ) to track the ground state energies. ( b ) Expected energy spectrum for the first shell of electrons and holes including the spin-orbit interaction. ( c , d ) Magnetic field dependence of line cuts in gate space (white dashed lines in a ) for the first two electrons, ( c ), and holes, ( d ). Coloured circles indicate positions on the corresponding bias triangles in ( a ), and the dashed lines indicate the observed magnetic field dependence of the ground states, in good agreement with the spin-orbit spectrum, ( b ). High magnetic field slopes for the ground state energies are indicated in the figures. We extract spin-orbit splittings meV for the first electron shell and meV for the first hole shell. Excited states inside the bias triangles (colour scale data above dashed lines) exhibit a rich structure as a function magnetic field, which we discuss elsewhere [33] . Full size image From the slopes of the ground states, we predict that first two electron levels will cross at a magnetic field B 2 =Δ SO / gμ B =15 T, while the first two hole levels do not cross. The crossing of the first two electron levels instead of the hole states, as was observed by Kuemmeth et al. [8] , implies the opposite sign of the spin-orbit interaction, likely due to a different chirality of our nanotube. The absence of the low Dirac-field crossing, however, does not allow us to clearly separate the orbital and Zeeman contributions, as was possible for the other two devices. We have observed strong spin-orbit couplings in carbon nanotubes that are an order of magnitude larger than that predicted by theory, with splittings up to Δ SO =3.4 meV. By using a low Dirac field, we are able to identify a strong Zeeman-type coupling in two devices. The origin of the large magnitude of the spin-orbit splitting observed remains an open question. Nonetheless, the observed strength of the coupling is promising for many applications of the spin-orbit interaction in carbon nanotube devices. Sample fabrication The devices are made using a fabrication technique in which the nanotube is deposited in the last step of the fabrication. Single quantum dot devices were fabricated by growing the device across predefined structures with three gates, using W/Pt electrodes for electrical contacts to the nanotube, and a dry-etched doped silicon layer to make gates [23] . Double quantum dot devices were fabricated by growing the nanotube on a separate chip [33] . Measurements Measurements were performed with a base electron temperature of 100 mK. For measurements performed with single quantum dot devices, a magnetic field was applied with an orientation in the plane of the sample, perpendicular to the trench. In measurements with double quantum dot devices, a 3D vector magnet was used to align the direction of the magnetic field along the axis of the nanotube. The measurement data sets presented in this manuscript are available online, see Supplemenatary Data 1 . Extraction of the ground state energies In order to convert changes in gate voltage position of the Coulomb peak to changes in energy of the ground state, a scaling factor α is required that converts gate voltage shifts into an energy scale. This scaling factor is measured by the lever-arm factor from the Coulomb diamond data, such as that shown in Supplemenatary Fig. S3 . In addition to the scaling of gate voltage to energy, the ground state magnetic field dependence traces must be offset by an appropriate amount, corresponding to subtracting the Coulomb energy from the addition energy, to produce spectra such as that shown in Fig. 3 of the main text. To determine this offset, we use the fact that at B =0, time-reversal symmetry requires that the electron states are two-fold degenerate. The offset for the 1e/2e curves was thus chosen such that the extrapolated states are degenerate at B =0. This was also used to determine the offset between the 3e/4e curves. For the remaining offset between the 2e and 3e curves, we use the level crossing that occurs at B 1 . At B 1 , the levels may exhibit a splitting due to intervalley scattering. This results in a ground state energy, which does not show a sharp kink at B 1 , but instead becomes rounded. The rounding of this kink in our data, however, is small. We estimate Δ KK ~0.1 meV, and have offset the 2e/3e curves by this amount at the crossing at B 1 . The spin-orbit splittings are determined by the zero-field gap in the resulting ground-state spectra. The error bars quoted on the spin-orbit splittings are estimates based on the accuracy with which the ground states energy curves can be aligned to produced plots such as those in Fig. 3 of the main text. How to cite this article: Steele, G.A. et al. Large spin-orbit coupling in carbon nanotubes. Nat. Commun. 4:1573 doi: 10.1038/ncomms2584 (2013).